Regulation of endogenous transmembrane receptors through optogenetic Cry2 clustering Transmembrane receptors are the predominant conduit through which cells sense and transduce extracellular information into intracellular biochemical signals. Current methods to control and study receptor function, however, suffer from poor resolution in space and time and often employ receptor overexpression, which can introduce experimental artefacts. We report a genetically encoded approach, termed Cl ustering I ndirectly using Cr yptochrome 2 (CLICR), for spatiotemporal control over endogenous transmembrane receptor activation, enabled through the optical regulation of target receptor clustering and downstream signalling using noncovalent interactions with engineered Arabidopsis Cryptochrome 2 (Cry2). CLICR offers a modular platform to enable photocontrol of the clustering of diverse transmembrane receptors including fibroblast growth factor receptor (FGFR), platelet-derived growth factor receptor (PDGFR) and integrins in multiple cell types including neural stem cells. Furthermore, light-inducible manipulation of endogenous receptor tyrosine kinase (RTK) activity can modulate cell polarity and establish phototaxis in fibroblasts. The resulting spatiotemporal control over cellular signalling represents a powerful new optogenetic framework for investigating and controlling cell function and fate. Cells receive dynamic information via transmembrane receptor signals and integrate these cues to regulate diverse biological processes including cell proliferation, motility, differentiation and death. Currently utilized approaches to study transmembrane receptor signalling [1] , [2] often employ overexpression of receptors and receptor fusions, which fundamentally alter how cells respond to extracellular signals and frequently induce hypersensitive or constitutive signal activation [3] , [4] , [5] . Indeed, receptor gene amplification and overexpression is a common driving factor of cancer cell transformation [6] , [7] . Moreover, current approaches do not provide a high degree of temporal and spatial control that would be desirable to study receptor signalling dynamics and spatially heterogeneous behaviour, respectively. In recent years, the emerging field of optogenetics has offered several methods to optically control and study numerous signalling phenomena with spatiotemporal precision [8] , [9] , [10] , [11] , [12] , [13] , [14] , [15] , [16] , [17] , although each currently relies on the ectopic expression of the signalling protein of interest. In a recent example, we co-opted the inherent blue-light-dependent oligomerization of Arabidopsis Cry2 to regulate clustering and activation of fusion proteins in the cytosol of mammalian cells [16] . In this report, we demonstrate the optogenetic control of endogenous transmembrane receptor activity. Our approach makes use of receptor clustering, which is a natural mechanism of activation for many important transmembrane receptors, including receptor tyrosine kinases, immune receptors (for example, T-cell receptor (TCR), B-cell receptor (BCR) and Fc receptor (FcR)), Wnt receptors and integrins [18] , [19] , [20] , [21] , [22] , [23] , [24] , [25] , [26] . Specifically, we re-designed and implemented Cry2 clustering to optically target, cluster and regulate endogenous transmembrane proteins in a modular strategy called Cl ustering I ndirectly using Cr yptochrome 2, or CLICR. CLICR design In designing CLICR ( Fig. 1a ), we hypothesized that Cry2 fused to a binding domain (Cry2-BD) possessing limited affinity for a target receptor would remain largely in the cytoplasm in the absence of light. On blue light illumination, clusters of Cry2-BD would assemble and thereby effectively create high local concentrations of the BD that may enable simultaneous binding to multiple receptor endodomains, resulting in receptor clustering and signal activation. 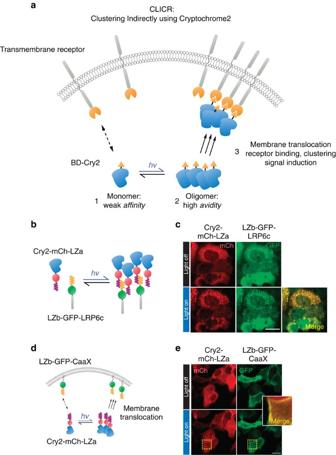Figure 1: The CLICR strategy enables Cry2 activation of transmembrane receptors. (a) CLICR allows modular Cry2 clustering and activation of membrane receptors via noncovalent interactions, avoiding complications associated with overexpression of receptor fusions. With CLICR, Cry2 fused to a receptor-targeting binding domain (BD) is expressed in the cytoplasm. In the dark, unclustered state, BD affinity for the receptor is weak and imparts no or little membrane localization. On light-induced clustering, BD-Cry2 oligomers increase local BD concentration, enabling membrane translocation, binding and nucleation of a receptor cluster. (b) CLICR allows clustering of cytoplasmic protein targets. On light activation, the Cry2-mCh-LZa (red) and LZb-GFP-LRP6c (green) components co-cluster (c), suggesting successful clustering of noncovalently bound proteins via homo-oligomerization of Cry2. (d,e) CLICR clustering also enables membrane translocation of the initially cytoplasmic Cry2-mCh-LZa. Scale bars, 20 μm. Figure 1: The CLICR strategy enables Cry2 activation of transmembrane receptors. ( a ) CLICR allows modular Cry2 clustering and activation of membrane receptors via noncovalent interactions, avoiding complications associated with overexpression of receptor fusions. With CLICR, Cry2 fused to a receptor-targeting binding domain (BD) is expressed in the cytoplasm. In the dark, unclustered state, BD affinity for the receptor is weak and imparts no or little membrane localization. On light-induced clustering, BD-Cry2 oligomers increase local BD concentration, enabling membrane translocation, binding and nucleation of a receptor cluster. ( b ) CLICR allows clustering of cytoplasmic protein targets. On light activation, the Cry2-mCh-LZa (red) and LZb-GFP-LRP6c (green) components co-cluster ( c ), suggesting successful clustering of noncovalently bound proteins via homo-oligomerization of Cry2. ( d , e ) CLICR clustering also enables membrane translocation of the initially cytoplasmic Cry2-mCh-LZa. Scale bars, 20 μm. Full size image As Cry2 optogenetic clustering had been well characterized using cytoplasmic proteins [16] , we first assessed the feasibility of CLICR by investigating whether we could optically cluster a Cry2-binding target in the cytoplasm and whether indirect clustering could induce signal activation ( Fig. 1b , Supplementary Fig. 1 ). Using a heterodimeric pair of leucine zippers [27] , we grafted one of the LZ helices (LZa) on the Cry2 module fused to mCherry (mCh) and its partner helix (LZb) on a green fluorescent protein (GFP)–LRP6c fusion, whose clustering has been shown to robustly stimulate the β-catenin pathway signalling [16] , [28] . A list of fusion architectures examined can be found in Supplementary Table 1 , and a complete list of constructs generated for this work can be found in Supplementary Data 1 . On co-transfection of the LZ-appended Cry2 and LRP6c fusions into HEK 293T cells, we observed light-induced cluster formation in both the mCherry and GFP channels, and these clusters colocalized, suggesting that Cry2 clusters were successfully clustering GFP–LRP6c fusions via the LZa–LZb interaction ( Fig. 1c , Supplementary Fig. 1b ). Cytoplasmic and membrane-targeted signal activation through CLICR To determine whether the light-stimulated LRP6c clusters were sufficient to induce β-catenin signalling, we transfected combinations of Cry2- and LRP6c-containing fusion pairs into 293T cells harbouring a β-catenin-responsive luciferase reporter [29] ( Fig. 1c ). Significant increases in β-catenin signalling in illuminated versus unilluminated samples were observed with all Cry2/LRP6c fusion pairs tested, although this signal was markedly diminished compared with that obtained with a single-chain Cry2-mCh-LRP6c fusion ( Supplementary Fig. 1d ) [16] , potentially because of LRP6c cluster geometries, expression level differences or differences in efficiencies of two-component versus one-component clustering. We further demonstrated the feasibility and modularity of the CLICR approach by indirectly clustering the Rac1 GTPase with the same LZ-binding adapters ( Supplementary Fig. 1e ). Consistent with our previous report of clustering the Rac1 protein [16] , indirect Rac1 clustering induced rapid membrane translocation of the Rac1 (and associated Cry2) fusion ( Supplementary Fig. 1f ). Together, the LRP6c and Rac1 results demonstrate that CLICR can serve as a modular strategy for clustering binding partners via noncovalent interactions. We next investigated whether a CLICR-induced avidity increase was sufficient to elicit translocation of a cytoplasmic Cry2 fusion to the plasma membrane, which would be necessary for CLICR activation of membrane receptors ( Fig. 1a ). We co-transfected cells with a membrane-localized LZb–GFP–CaaX construct, which is lipid-modified at the C-terminal CaaX box, and Cry2-fused to mCherry with the LZa helix at either the C- or N terminus ( Fig. 1d , Supplementary Fig. 2a ). In the dark state, LZb–GFP–CaaX appeared membrane-bound, whereas Cry2–LZa fusions were largely cytoplasmic with few regions of visible membrane association, suggesting weak basal affinity of the LZa–LZb binding partners. On light illumination, both Cry2 fusions exhibited translocation to the cell periphery and to immobilized puncta within the cell body, suggesting strong light-induced binding to cell membranes ( Fig. 1e , Supplementary Fig. 2b ). To analyse whether CLICR-mediated membrane translocation could induce signalling on binding and clustering of a transmembrane receptor, we replaced the LZb–GFP–CaaX fusion with a GFP–LZb fused to the C terminus of the full-length LRP6 receptor ( Supplementary Fig. 3a ), whose clustering induces β-catenin signalling [28] . LRP6–GFP–LZb was localized to multiple cellular compartments ( Supplementary Fig. 3b ), and illumination of Cry2 with N- or C-terminally fused LZa ( Supplementary Fig. 3c,d ), but not with Cry2 lacking the LZa ( Supplementary Fig. 3e,f ), successfully induced Cry2 translocation and colocalization with LRP6–GFP–LZb as well as activation of the β-catenin luciferase reporter, although high background signal was observed in the dark ( Supplementary Fig. 3g ) because of receptor overexpression ( Supplementary Fig. 3h ). By comparison, a direct LRP6–Cry2 fusion resulted in a constitutive signal that could not be further enhanced by illumination, further representative of artefact that can accompany overexpression of transmembrane receptor constructs ( Supplementary Fig. 4 ). These results both provided support for the CLICR approach and motivated adapting it to activate endogenous receptors and thus overcome overexpression artefact. Targeting of receptor tyrosine kinases The receptor tyrosine kinase (RTK) class of receptors is broadly important in regulating proliferation, growth, differentiation, survival and motility, and activation of many RTKs involves lateral interactions including clustering [23] . Furthermore, signalling artefacts are commonly observed on RTK overexpression within cells [3] , [5] . To target a cell’s native RTKs with CLICR, we used the N-terminal src-homology 2 (SH2) domain from PLC-γ as our binding domain adapter ( Fig. 2a ). Since the SH2 domain typically does not bind unphosphorylated peptide sequences, we hypothesized that SH2 domain clustering may enhance its avidity for unactivated or weakly activated receptors [30] and subsequently cluster and activate the RTKs. To test RTK-targeting ability, we expressed mCherry-Cry2 with an N-terminal SH2 domain (SH2-N) in several cell types, including HEK 293Ts, 3T3 fibroblasts and adult neural stem cells (NSCs). In 293Ts, illumination of SH2-N yielded membrane-anchored puncta ( Fig. 2b , top row; Supplementary Movie 1 ). Analogously, 3T3 fibroblasts exhibited rapid localization of SH2-N to membrane-anchored puncta as well as to focal adhesion structures ( Fig. 2c , top row, Supplementary Movie 2 ), and NSCs exhibited light-induced punctate formation in neurite extensions as well as in the cell body, collectively suggesting that SH2-N may target endogenous membrane proteins ( Fig. 2d , top row; Supplementary Movie 3 ). A C-terminal fusion of SH2 to Cry2-mCh (SH2-C) was also tested and yielded similar phenotypes, although with slower kinetics, and the SH2-N construct was thus used for all further experiments. Treatment with the RTK inhibitor PD-089828 (RTKi)—which inhibits phosphorylation of the RTKs FGFR1, PDGFRβ and EGFR—markedly reduced SH2-N focal enrichment at the membrane in all three cell types ( Fig. 2b–d , bottom rows). These data indicate that strong SH2-N localization is dependent on RTK phosphorylation, and thus SH2-N clusters are indeed targeting endogenous RTK receptors. 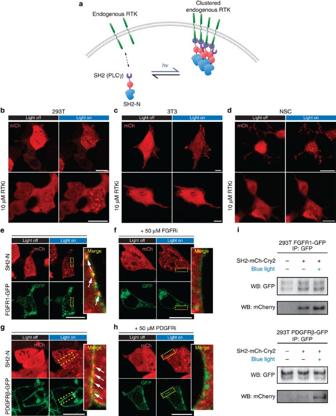Figure 2: CLICR can target and cluster endogenous transmembrane receptors. (a) To target endogenous receptors with CLICR, an adapter domain with affinity for native receptors was used in place of the engineered LZa–LZb interaction used previously. The SH2 domain from PLCγ was used as a binding domain fused to the N terminus of mCh-Cry2 (SH2-N) to target endogenous receptor tyrosine kinases. Illuminated SH2-N expressed in 293Ts (b, top panels) localized to membrane-anchored foci. In 3T3 fibroblasts (c, top panels), illumination of SH2-N induced translocation to the membrane periphery and to structures resembling focal adhesions. In NSCs (d, top panels), illuminated SH2-N localized to immobilized membrane clusters both in the cell body and in neurites. In all three cell types, inhibition with an FGFR1/PDGFRβ/EGFR-specific inhibitor (RTKi) largely abrogated visible SH2-N translocation. (b–d, lower panels). In 293Ts, upon blue light illumination SH2-N colocalized (arrows) to exogenously expressed, full-length FGFR1 (e) and PDGFRβ (g) fused to GFP, and this colocalization was abrogated in the presence of inhibitors specific to these receptors (f,h). Scale bars, 20 μm. Light-stimulated association of SH2-N with either FGFR1-GFP or PDGFRβ-GFP was confirmed through co-immunoprecipitation of SH2-N with the receptors (i). Figure 2: CLICR can target and cluster endogenous transmembrane receptors. ( a ) To target endogenous receptors with CLICR, an adapter domain with affinity for native receptors was used in place of the engineered LZa–LZb interaction used previously. The SH2 domain from PLCγ was used as a binding domain fused to the N terminus of mCh-Cry2 (SH2-N) to target endogenous receptor tyrosine kinases. Illuminated SH2-N expressed in 293Ts ( b , top panels) localized to membrane-anchored foci. In 3T3 fibroblasts ( c , top panels), illumination of SH2-N induced translocation to the membrane periphery and to structures resembling focal adhesions. In NSCs ( d , top panels), illuminated SH2-N localized to immobilized membrane clusters both in the cell body and in neurites. In all three cell types, inhibition with an FGFR1/PDGFRβ/EGFR-specific inhibitor (RTKi) largely abrogated visible SH2-N translocation. ( b – d , lower panels). In 293Ts, upon blue light illumination SH2-N colocalized (arrows) to exogenously expressed, full-length FGFR1 ( e ) and PDGFRβ ( g ) fused to GFP, and this colocalization was abrogated in the presence of inhibitors specific to these receptors ( f , h ). Scale bars, 20 μm. Light-stimulated association of SH2-N with either FGFR1-GFP or PDGFRβ-GFP was confirmed through co-immunoprecipitation of SH2-N with the receptors ( i ). Full size image To further validate that SH2-N was binding RTKs, we transfected the SH2-N construct into 293Ts stably expressing GFP-tagged, full-length FGFR1 or PDGFRβ receptors, representing two RTKs that bind the PLCγ SH2 domain [31] , [32] . In cells expressing ectopic FGFR1–GFP, the SH2-N construct exhibited light-dependent membrane translocation and formation of puncta that colocalized with GFP ( Fig. 2e ). Addition of 50 μM FGFR1–4 inhibitor (PD-166866, FGFRi) abrogated this colocalization ( Fig. 2f ). Similar behaviour was obtained in cells expressing PDGFRβ-GFP, where light-induced SH2-N colocalization with PDGFRβ-GFP ( Fig. 2g ) was abrogated in the presence of 50 μM PDGFR-α and -β inhibitor (CAS 205254-94-0, PDGFRi; Fig. 2h ). Light-promoted SH2-N binding to FGFR1 and PDGFRβ was further established through co-immunoprecipitation of SH2-N with either the FGFR1 or PDGFRβ receptors ( Fig. 2i ). Together, these results indicate that the cytoplasmic SH2-N construct can successfully target native transmembrane RTKs via CLICR in response to light. Optogenetic activation of endogenous transmembrane receptors We next investigated whether SH2-based CLICR targeting of endogenous RTKs is capable of signal activation. Illumination of 3T3 fibroblasts expressing SH2-N yielded a broad increase in tyrosine phosphorylation, compared with unilluminated and RTKi-inhibited controls ( Fig. 3a ). Furthermore, analysis of canonical RTK signalling pathways showed an increase in levels of phospho-Akt and phospho-Erk1/2 after 15 min of blue light illumination, a difference abrogated in the presence of the RTKi inhibitor. A central benefit of employing CLICR for RTK activation is the lack of receptor overexpression, which may introduce artefacts including hypersensitity to extracellular ligand. Indeed, in contrast to cells overexpressing a PDGFRβ–Cry2 fusion, SH2-N-expressing cells retained native sensitivity to extracellular PDGF-BB ( Supplementary Fig. 6 ). 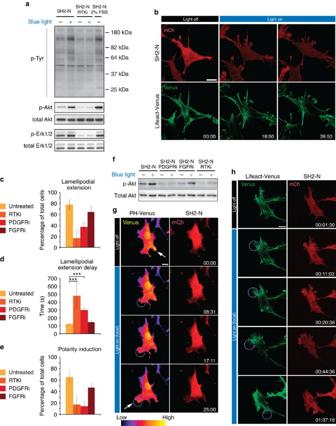Figure 3: CLICR allows photoactivation of endogenous RTKs in fibroblasts and enables PDGFRβ-dependent phototaxis. Western blot analysis (a) of serum-starved fibroblasts treated for 10 min with blue light shows broad upregulation of tyrosine phosphorylation in illuminated versus unilluminated samples, and this difference is abrogated by 10 μM RTKi treatment. Samples grown in 2% serum were used as a positive control. In particular, light-treated samples demonstrated an RTK-dependent increase in Akt and Erk1/2 phosphorylation. (b) Time-lapse imaging of SH2-N-expressing fibroblasts shows lamellipodial extension and cell repolarization upon whole-field blue light exposure. (c) The proportion of cells extending lamellipodia in response to whole-field illumination was reduced by broad RTK or PDGFR inhibition, but not FGFR inhibition. Error bars represent 95% confidence intervals,n=24–83 cells per condition. (d) Among cells extending light-induced lamellipodia under broad RTK inhibition or PDGFR inhibition, a longer delay before initial lamellipodial extension was evident, while FGFR inhibition did not induce a delay in extension. Graph shows means±1 s.d.,n=4–58 cells per condition. ***P<0.001 by one-way ANOVA with Tukey pairwise analysis. (e) The proportion of cells exhibiting light-induced polarization was reduced by the RTKi or PDGFRi treatment, and slightly reduced by FGFRi treatment. Error bars represent 95% confidence intervals,n=24–83 cells per condition. (f) Western blot analysis shows that illuminated SH2-N expressing cells exhibit Akt activation under mock and FGFRi treatment. PDGFRi and RTKi treatment abrogate Akt activation. (g) Focal illumination enabled the spatial definition of the lamellipodial extension region coupled with re-establishment of a PIP3 gradient at the site of illumination (arrows), as observed through a PH(Akt)-Venus biosensor. (h) CLICR-enabled focal activation of lamellipodial extension and polarity establishment allows the effective rewiring of PDGFR-dependent chemotaxis to respond to light. Fibroblasts co-expressing SH2-N and Lifeact-Venus were illuminated focally, and actin polymerization, lamellipodial extension and cell motility were induced in the direction of the illuminated region. Illuminating the trailing edge-induced re-polarization and a reversal of migration direction. Scale bars, 20 μm. To enhance visualization, excitation laser intensity was increased in bottom panels to compensate for photobleaching. Figure 3: CLICR allows photoactivation of endogenous RTKs in fibroblasts and enables PDGFRβ-dependent phototaxis. Western blot analysis ( a ) of serum-starved fibroblasts treated for 10 min with blue light shows broad upregulation of tyrosine phosphorylation in illuminated versus unilluminated samples, and this difference is abrogated by 10 μM RTKi treatment. Samples grown in 2% serum were used as a positive control. In particular, light-treated samples demonstrated an RTK-dependent increase in Akt and Erk1/2 phosphorylation. ( b ) Time-lapse imaging of SH2-N-expressing fibroblasts shows lamellipodial extension and cell repolarization upon whole-field blue light exposure. ( c ) The proportion of cells extending lamellipodia in response to whole-field illumination was reduced by broad RTK or PDGFR inhibition, but not FGFR inhibition. Error bars represent 95% confidence intervals, n =24–83 cells per condition. ( d ) Among cells extending light-induced lamellipodia under broad RTK inhibition or PDGFR inhibition, a longer delay before initial lamellipodial extension was evident, while FGFR inhibition did not induce a delay in extension. Graph shows means±1 s.d., n =4–58 cells per condition. *** P <0.001 by one-way ANOVA with Tukey pairwise analysis. ( e ) The proportion of cells exhibiting light-induced polarization was reduced by the RTKi or PDGFRi treatment, and slightly reduced by FGFRi treatment. Error bars represent 95% confidence intervals, n =24–83 cells per condition. ( f ) Western blot analysis shows that illuminated SH2-N expressing cells exhibit Akt activation under mock and FGFRi treatment. PDGFRi and RTKi treatment abrogate Akt activation. ( g ) Focal illumination enabled the spatial definition of the lamellipodial extension region coupled with re-establishment of a PIP3 gradient at the site of illumination (arrows), as observed through a PH(Akt)-Venus biosensor. ( h ) CLICR-enabled focal activation of lamellipodial extension and polarity establishment allows the effective rewiring of PDGFR-dependent chemotaxis to respond to light. Fibroblasts co-expressing SH2-N and Lifeact-Venus were illuminated focally, and actin polymerization, lamellipodial extension and cell motility were induced in the direction of the illuminated region. Illuminating the trailing edge-induced re-polarization and a reversal of migration direction. Scale bars, 20 μm. To enhance visualization, excitation laser intensity was increased in bottom panels to compensate for photobleaching. Full size image We further investigated whether CLICR clustering of the PLCγ SH2 domain demonstrated selectivity towards individual receptors. Since activated PDGFRβ has been shown to colocalize with focal adhesions through interaction with focal adhesion kinase [33] , we hypothesized that endogenous PDGFRβ activation was largely responsible for the CLICR-induced signal activation and focal adhesion translocation of SH2-N in our study ( Fig. 2c ). To address this possibility, we examined the light-induced translocation of SH2-N in the presence of pathway-specific inhibitors. In 3T3 fibroblasts, SH2-N exhibited a rapid, light-induced localization to the plasma membrane and focal adhesion structures. Moreover, the 10-μM PDGFRi treatment largely inhibited focal adhesion translocation of SH2-N ( Supplementary Fig. 5 ), whereas 10-μM FGFRi had minimal observed effect on focal SH2-N localization, suggesting that translocation was indeed PDGFRβ-dependent and that CLICR clustering was modulating PDGFRβ activity. In general, activated PDGFR colocalization with FAK within focal adhesions has been shown to modulate FAK activation, focal adhesion turnover and cell migration [34] . In addition, PDGFRβ-induced membrane recruitment of phosphatidylinositol-3-kinase (PI3K) leads to conversion of phosphatidylinositol-4,5-bisphosphate (PIP2) to phosphatidylinositol-3,4,5-trisphosphate (PIP3) [35] , whose localization at the leading edge of cells is a key factor in cellular polarity establishment and PDGFR-dependent fibroblast migration. We found that in fibroblasts, SH2-N translocation was accompanied by filopodial and lamellipodial extension, often followed by cellular polarization and movement ( Fig. 3b , Supplementary Movie 4 ). This polarization was dependent on PI3K activity, since addition of the PI3K inhibitor wortmannin led to only transient lamellipodial extensions ( Supplementary Fig. 6a , Supplementary Movie 5 ), which then rapidly stopped protruding or collapsed. PI3K activity was thus required to sustain membrane extensions and establish morphological polarity, consistent with CLICR-mediated activation of PDGFRβ and PI3K. We next quantified these PDGFR- and PI3K-dependent effects. Lamellipodial extension induced by whole-field illumination was observed in 78% of cells expressing SH2-N, and RTKi inhibition significantly reduced this response to 17% of cells ( Fig. 3c , with significance determined through nonoverlapping 95% confidence intervals). Likewise, PDGFRi significantly decreased the number of cells extending light-induced lamellipodia from 78 to 37%. In contrast, FGFRi had no effect on cell morphological responses. In cells that did exhibit lamellipodial response, we quantified the time interval from the start of blue light exposure to the first apparent lamellipodial extension. Untreated cells extended initial lamellipodia with an average interval of 123 s, while RTKi or PDGFRi significantly delayed such lamellipodial extension in responding cells to 481 and 300 s, respectively ( Fig. 3d , analysis of variance (ANOVA) with Tukey post hoc analysis, P <0.0001). In contrast, FGFRi treatment had no apparent effect on lamellipodial extension timing. We then examined the fraction of cells that established polarity and initiated migration on light treatment, as observed by inspecting lamellipodial extension coupled with trailing edge retraction and morphological reorientation. Sixty-five percent of uninhibited fibroblasts exhibited polarity establishment, and this response was significantly suppressed to 17 and 12% of cells treated with RTKi and PDGFRi, respectively ( Fig. 3e , significance determined through nonoverlapping 95% confidence intervals). By comparison, FGFRi treatment only moderately reduced light-dependent polarity induction (47% of cells). These results were further corroborated through western blotting, as light-induced Akt activity was observed in uninhibited and FGFRi-inhibited cells, but was absent in RTKi- and PDGFRi-inhibited cells ( Fig. 3f ). Collectively, although not demonstrating unique specificity of receptor targeting, these data demonstrate the ability of SH2-N to modulate endogenous PDGFRβ activation within 3T3 fibroblasts. Since PDGFRβ is a key mediator of fibroblast chemotaxis [36] , we next sought to exploit the spatiotemporal precision of CLICR and rewire a cell’s chemotactic circuitry to regulate migration in response to a light signal instead of a chemical one. We hypothesized that focal blue light illumination would establish and define a local PIP3 gradient, and that this would allow directed polarization, actin polymerization and motility of the cell. In fibroblasts co-expressing SH2-N and PH-Venus, which comprises Venus fused to the pleckstrin homology (PH) domain of Akt and is an established biosensor of PIP3 production [37] , the PH-Venus was initially inhomogeneously distributed, indicating initial polarization of PIP3 within the cell. Illuminating the cell in a region not exhibiting initially high levels of PIP3-induced membrane ruffling and lamellipodial extension towards the illumination region, coupled with a redistribution of PH-Venus ( Fig. 3g , Supplementary Movie 6 ). In particular, the extending lamellipodium exhibited high levels of PH-Venus recruitment, and within minutes the cell began moving towards the light, establishing a PIP3 gradient and a new leading edge as defined by the illumination region ( Fig. 3g , Supplementary Movie 6 ). In the presence of the PI3K inhibitor wortmannin, however, focal illumination was unable to induce the sustained extension of the illuminated region and establishment of a PIP3 gradient, confirming that local PIP3 production, polarization and motility were PI3K-dependent ( Supplementary Fig. 6b , Supplementary Movie 7 ). In addition, focal blue light illumination of SH2-N cells co-expressing a Lifeact-Venus probe for F-actin stimulated initial lamellipodial actin polymerization, membrane ruffling and extension within 30 s along with a coordinated initiation of trailing edge retraction ( Fig. 3h , Supplementary Movie 8 ). The cell proceeded to phototax in the direction of the initial illumination region until the light stimulus was reoriented, at which point the established lamellipodium collapsed, and the cells repolarized to migrate in the newly defined direction ( Fig. 3h , Supplementary Movie 8 ). CLICR can target diverse transmembrane receptors Finally, to demonstrate that CLICR may be a highly modular method for regulating diverse endogenous pathways, we devised a method to target β-integrin receptors, which participate in cellular adhesion complexes in their active state and can diffuse freely in the membrane in an inactive state. The important role of clustering in integrin affinity and activation [38] , [39] , [40] renders endogenous integrins attractive CLICR targets. For the binding adapter, we used the phosphotyrosine-binding-like F3 domain from talin, which binds β3-integrin cytoplasmic tails [41] and whose expression in a Cry2 fusion yielded no observed impact on basal cell signalling ( Supplementary Fig. 8 ). Co-immunoprecipitation of F3-mCh-Cry2 (F3-N) fusion with a co-expressed integrin-β3–GFP fusion revealed a strong light-dependent association, suggesting that F3 may be used as a binding adapter for targeting integrin-β3 clustering ( Fig. 4a ). Illumination of F3-N in fibroblasts yielded rapid punctate formation and notable motion of the induced puncta along defined intracellular trajectories ( Fig. 4b , Supplementary Movie 9 ). These phenotypic results were distinct from those described for SH2-N and were absent in cells expressing mCherry-Cry2 without the F3 domain ( Fig. 4b ). 3T3 cells co-expressing both F3-N and integrin-β3 revealed strong co-clustering of the two constructs under light illumination, with a reversion to diffuse localization in the dark ( Fig. 4c ). This co-clustering was observed in all 116 co-expressing cells in which the F3-N construct exhibited cluster formation ( Fig. 4d ). Furthermore, analysis of over 400 clusters within cytoplasmic regions of these cells revealed that every F3-N cluster colocalized with an integrin-β3 cluster ( Fig. 4e,f ), suggesting a strong ability for the F3 domain to enable integrin-β3 clustering via CLICR and overall demonstrating the generality of the CLICR approach for targeting diverse membrane targets [42] . 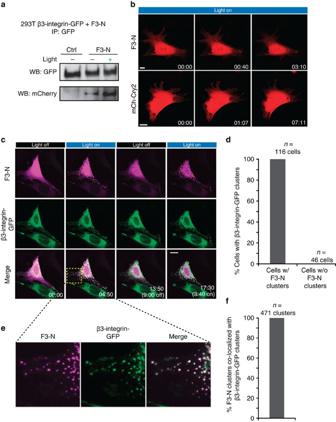Figure 4: CLICR targeting and clustering of β-integrins. (a) Co-immunoprecipitation of the talin F3 domain fused to mCh-Cry2 (F3-N) co-expressed with integrin-β3-GFP in HEK 293T cells reveals strong association of the constructs under blue light exposure. (b) Fibroblasts expressing F3-N show light-induced formation of puncta that move within the cell along defined linear trajectories (seeSupplementary Movie 9). (c) Co-expression of F3-N and integrin-β3-GFP in 3T3 cells demonstrates a high degree of co-clustering of the two constructs under blue light, with reversion of clusters to a diffuse state in the dark. (d) All co-expressing cells incthat displayed F3-N clustering exhibited concomitant β3-integrin co-clustering. Further analysis of quantifiable cellular regions (e) revealed that all observable F3-N clusters co-clustered with integrin-β3-GFP (f). Scale bars, 20 μm. Figure 4: CLICR targeting and clustering of β-integrins. ( a ) Co-immunoprecipitation of the talin F3 domain fused to mCh-Cry2 (F3-N) co-expressed with integrin-β3-GFP in HEK 293T cells reveals strong association of the constructs under blue light exposure. ( b ) Fibroblasts expressing F3-N show light-induced formation of puncta that move within the cell along defined linear trajectories (see Supplementary Movie 9 ). ( c ) Co-expression of F3-N and integrin-β3-GFP in 3T3 cells demonstrates a high degree of co-clustering of the two constructs under blue light, with reversion of clusters to a diffuse state in the dark. ( d ) All co-expressing cells in c that displayed F3-N clustering exhibited concomitant β3-integrin co-clustering. Further analysis of quantifiable cellular regions ( e ) revealed that all observable F3-N clusters co-clustered with integrin-β3-GFP ( f ). Scale bars, 20 μm. Full size image Spatially defined and rapidly time-varying signals are the key regulatory factors in diverse biological processes including cell migration [43] , asymmetric cell division [44] , differentiation [5] and apoptosis [45] . The difficulties of perturbing biological systems with such spatiotemporal precision, however, often preclude our understanding of how dynamic signals regulate cellular function. Optogenetic tools address this need. Although methods for optical protein homodimerization [15] , [46] , heterodimerization [11] , [12] , [13] , [14] and homo-oligomerization [16] of ectopically expressed proteins have been developed, ectopic expression of many signalling proteins—particularly transmembrane receptors—can fundamentally alter how the system of study behaves, potentially confounding conclusions reached with even the most sophisticated perturbative techniques. We devised the CLICR method to address this dilemma. The CLICR strategy provides a modular, single construct system to optically cluster and activate transmembrane receptors from the cytosol and is a powerful method for reversibly modulating endogenous transmembrane receptor activity. We accomplished this by pairing Cry2 clustering with a binding adapter for our target receptors. Although we envisioned the ideal CLICR adapter to have weak target affinity in the monomeric state and strong avidity on clustering, it is possible that the CLICR strategy would also work for adapters with strong target affinities. In this case, Cry2-BD would bind the target in the monomeric dark state, and light would induce clustering of these Cry2-BD:target complexes. Indeed, this would be analogous to activation of direct Cry2-receptor fusions [47] , [48] with the added benefit of targeting endogenous pools of signalling proteins. We note that we do anticipate some levels of basal (light-independent) interaction of our LZa–LZb-binding adapters in the dark state in Fig. 1 and Supplementary Figs 1–3 . Our ability to enhance these interactions and observe light-dependent phenotypes further suggests that CLICR can work for binding adapters with a range of binding affinities. We present CLICR here as a proof of concept strategy demonstrating the feasibility of targeting and activating endogenous receptor activity with light. Since the SH2-N and F3-N constructs bind endogenous phosphotyrosine sites and can therefore have an impact on and be subjected to the native regulation of those phosphorylation sites, we stress that the orthogonality and appropriateness of these and similar tools must be empirically validated for each system before use. Development of alternative, ‘orthogonal’ binding domains, for example an intracellular antibody domain specifically evolved to target a receptor endodomain [49] , may in the future offer additional versatility, specificity and reduction of basal signal perturbation. Studies should also include controls for Cry2 expression. Although it is unclear to what extent this plant protein domain interacts with mammalian cell machinery, at least one interaction has already been identified [50] . While our report was under revision, several studies that also further developed optogenetic Cry2 clustering were published. One group applied Cry2 homo-oligomerization for optogenetic activation of overexpressed receptors [47] , [48] . The demonstrated ability to apply this strategy to multiple RTKs makes this a powerful approach, although we again caution that receptor overexpression often leads to enhanced signalling artefacts ( Supplementary Figs 3h,g, 4 and 6 ), potentially altering the system of study. An additional study engineered Cry2 (Cry2-olig) [51] to form larger clusters than reported with wild-type Cry2 (ref. 16 ) and used this mutant to sequester and interfere with the function of endogenous proteins. This expansion of Cry2-clustering variants presents a choice for researchers based on their optogenetic needs. For studies seeking to sequester and inhibit protein function, large clusters with slow OFF-kinetics, such as those provided by Cry2-olig, may be ideal. For studies requiring temporally precise activation of endogenous proteins with low background activation, the weaker-associating wild-type Cry2 with faster OFF faster kinetics may be more appropriate. In sum, receptor overexpression can often elevate pathway signalling above the physiologically basal state and/or alter signal response dynamics. As an alternative, our demonstrated activity, modularity and versatility of CLICR across numerous cell types suggests its utility as an optogenetic tool to manipulate endogenous protein activity across biological systems. DNA vector assembly All vectors were constructed using the CPEC method [52] and through standard restriction enzyme cloning [16] . Full sequences and descriptions of all constructs used are provided in Supplementary Data 1 . The LZa and LZb heterodimeric leucine zipper pair corresponds to leucine zipper pair (vii), as described [27] , and was synthesized through primer overlap extension. We received the full-length LRP6 construct from Dr Xi He, the Rac1 construct from Dr G. Steven Martin, the Akt construct from Dr S. Ferguson, the PDGFR β, and 7x TCF constructs from Addgene (no. 23893 and no. 24308, respectively), and the PLC γ -1 construct from the DNASU plasmid repository (clone IDs HsCD00321979 and HsCD00435250, respectively). The FGFR1 construct was cloned from a rat NSC cDNA library. Cell culture, reagents, plasmid transfection and viral transduction HEK 293Ts were cultured in Dulbecco’s Modified Eagle Medium (DMEM, Corning Cellgro) with 10% fetal bovine serum (FBS; Life Technologies) and 1% penicillin/streptomycin (P/S; Life Technologies) at 37 °C and 5% CO 2 . NIH 3T3 fibroblasts were cultured in DMEM supplemented with 10% bovine calf serum and 1% P/S. Rat hippocampal adult NSCs [53] were cultured on polystyrene plates coated with poly-ornithine and 5 μg/ml laminin (Life Technologies), with DMEM/F12 (1:1) high-glucose medium containing N-2 supplement (both from Life Technologies) and 20 ng/ml recombinant human FGF-2 (Peprotech). Transient plasmid transfection was performed using the calcium phosphate method. Retroviral and lentiviral packaging and transduction were performed as described [54] . Briefly, VSVG-pseudotyped virus was packaged in 293T cells. Cell culture medium from virus-producing cells was collected on day 2 and day 3 post transfection, sterile-filtered, and purified through ultracentrifugation and resuspension in PBS. All retroviral constructs were based on the CLPIT retroviral vector and were packaged in the presence of 3 μg/ml doxycycline to repress transgene expression in order to maximize viral titre. RTKi (PD-089828), PDGFRi (CAS 205254-94-0, IC 50 =50 nM for PDGFR-β) and FGFRi (PD-166866, IC 50 =60 nM for FGFR1) were obtained from Millipore. Luciferase assay HEK 293T cells stably transduced with a 7 × Tcf luciferase reporter were seeded in black-walled 96-well plates. When ∼ 50% confluent, the cells were transfected with 5 ng of each expression vector diluted in 150 ng pBluescript. Cells were given 24 h to express protein and were then illuminated overnight for 16 h with one 500-ms pulse of light-emitting diode (LED) light every 10 s as administered by a custom LED illumination device [16] . After illumination, cells were lysed, and luciferase was measured with the Luc-screen Firefly Luciferase Gene Reporter System (Life Technologies). Confocal microscopy Time-lapse microscopy of activated Cry2 fusions was performed on a Zeiss LSM 710 AxioObserver confocal microscope with full incubation chamber in conjunction with the Zeiss ZEN software. Cry2 translocation experiments were carried out at 25 °C, while experiments examining cell motility and polarity were carried out at 37 °C and in 5% CO 2 . EGFP, Venus and mCherry were visualized with 488, 514 and 561 nm laser excitation, respectively, through either a × 40 or × 63 oil immersion objective. Whole-field Cry2 activation was achieved using 450- or 488-nm illumination. Spatially defined activation was carried out under whole-cell imaging of Venus with a 514-nm laser in conjuction with focal illumination using the FRAP application with 458- or 488-nm laser light at 1–5% power and 10 μs dwell time per pixel in a 10-μm diameter region. For whole-field observation of lamellipodial induction and polarity establishment, cells were excited every 13 s with 488-nm light, and mCherry was imaged simultaneously. Image analysis For whole-field observation of lamellipodial induction and polarity establishment, cells were simultaneously excited with 488-nm light and imaged for mCherry and Lifeact-Venus localization. Time-lapse image stacks were assembled in ImageJ, and each cell was examined for the appearance of new lamellipodia and for the time elapsed from the start of blue light excitation to initial lamellipodial appearance. To assess polarity establishment, cells were scored for the presence of lamellipodial formation coupled with visible trailing edge retraction and morphological reorientation. Western blotting 3T3s expressing SH2-N were seeded in 35-mm plates at 50% confluence and 2% FBS. After 24 h, the medium was exchanged, and cells were serum-starved for 16 h. Positive control cells remained in 2% serum. RTKi (10 μM) was added 30 min before illumination. Light-treated plates were illuminated with a 19 LED array (ledlight.com, cat. no. 28345) at 37 °C in a standard cell culture incubator with a 500-ms pulse every 2 s for 15 min. Cells were immediately lysed in cold RIPA buffer containing protease and phosphatase inhibitors, and were separated electrophoretically on a 10% SDS–PAGE gel. Proteins were then blotted on a nitrocellulose membrane and probed for phospho-Tyrosine (P-Tyr-1000, Cell Signaling no. 9411, 1:2,000 dilution), phospho-Akt (Cell Signaling no. 4060, 1:2,000 dilution), total Akt (Cell Signaling no. 9272, 1:1,000 dilution), phospho-Erk1/2 (Cell Signaling no. 4370, 1:2,000 dilution) and total Erk1/2 (Cell Signaling no. 4695, 1:1,000 dilution). For experiments examining signalling artefact, cells were seeded in 10% serum and starved overnight. Cells were then collected or stimulated with varying concentrations of PDGF-BB for 15 min before harvesting and performing SDS–PAGE and western blot. Phospho-serine (Abcam no. ab9332, 1:100 dilution), phospho-thereonine (Cell Signaling no. 9381, 1:1,000 dilution) and phospho-tyrosine (P-Tyr-1000, Cell Signaling no. 9411, 1:2,000 dilution) were used to assess phosphosignalling state. Uncropped images of the western blots are shown in Supplementary Fig. 9 . Immunoprecipitation 293Ts stably expressing full-length PDFGRβ-GFP or FGFR1-GFP were seeded in 10-cm plates. When ∼ 70% confluent, each plate was transfected with 1 μg 6xHis-SH2-mCh-Cry2 plasmid DNA diluted in 9 μg pBluescript by the calcium phosphate method. Twenty-four hours after transfection, cells were serum-starved overnight. Light-treated plates were illuminated with a 19-LED array for 10 min at 25 °C, after which cells were lysed in 1 ml RIPA buffer. After incubation on ice for 30 min, the cell lysate was spun at 4 °C for 10 min, and the supernatant from each sample was incubated with 5 μg of anti-GFP antibody (Life Technologies, A-11122). Antibody-lysate solutions were incubated overnight at 4 °C with gentle shaking and were then incubated in 12.5 μl immobilized protein A/G agarose beads (Thermo Scientific no. 20421) for 1 h as per the manufacturer’s instructions. Beads were spun down and washed with lysis buffer three times, followed by one final wash with water. Beads were then incubated in 2 × SDS sample buffer, boiled for 10 min, spun down one final time, separated via SDS–PAGE and blotted on a nitrocellulose membrane. Blots were then probed for GFP or mCherry (Clontech no. 632543, 1:1,000 dilution). Statistical methodology Statistical power in luciferase assays was determined through the nonparametric Mann–Whitney Wilcoxon test. For comparing lamellipodial extension delays, varying dosages for the RTKi and PDGFRi treatment were compared using one-way ANOVA followed by Tukey post hoc pairwise analysis, with a significance threshold adjusted using the Bonferroni correction. FGFRi inhibition was compared with untreated cells using a Student’s t -test. All statistical analyses were performed using the JMP statistical software suite. How to cite this article: Bugaj, L. J. et al . Regulation of endogenous transmembrane receptors through optogenetic Cry2 clustering. Nat. Commun. 6:6898 doi: 10.1038/ncomms7898 (2015).